Red fluorescent genetically encoded indicator for intracellular hydrogen peroxide Reactive oxygen species (ROS) are conserved regulators of numerous cellular functions, and overproduction of ROS is a hallmark of various pathological processes. Genetically encoded fluorescent probes are unique tools to study ROS production in living systems of different scale and complexity. However, the currently available recombinant redox sensors have green emission, which overlaps with the spectra of many other probes. Expanding the spectral range of recombinant in vivo ROS probes would enable multiparametric in vivo ROS detection. Here we present the first genetically encoded red fluorescent sensor for hydrogen peroxide detection, HyPerRed. The performance of this sensor is similar to its green analogues. We demonstrate the utility of the sensor by tracing low concentrations of H 2 O 2 produced in the cytoplasm of cultured cells upon growth factor stimulation. Moreover, using HyPerRed we detect local and transient H 2 O 2 production in the mitochondrial matrix upon inhibition of the endoplasmic reticulum Ca 2+ uptake. Oxygen is a central molecule of aerobic life serving not only as a terminal acceptor of electrons in the respiratory chain but also as a global regulator of many physiological and pathological processes. This regulation is mostly mediated by reactive oxygen species (ROS) that are physiologically produced in a cell in a tightly controlled manner. Uncontrolled production of ROS under pathological conditions leads to a non-specific damage of proteins, lipids and DNA, known as oxidative stress [1] , [2] . The primary reactive oxygen intermediate is the superoxide anion radical O 2 · − (superoxide), which is produced by many enzymatic systems by one-electron oxygen reduction. Superoxide rapidly undergoes dismutation to hydrogen peroxide, a relatively stable molecule with high reaction specificity towards deprotonated Cys residues (thiolates) [3] . Reversible oxidation of thiolates by H 2 O 2 is a central molecular mechanism underlying so-called ‘redox signalling’ [4] . As many proteins in the cell contain redox-active thiolates in catalytically active centres or allosteric sites, controlled production of H 2 O 2 enables precise redox regulation of various cellular metabolic pathways and signalling cascades. Recent progress in probe development has enabled imaging of H 2 O 2 in complex systems. A number of genetically encoded and synthetic H 2 O 2 indicators have been designed and tested in vitro and in vivo [5] , [6] , [7] , [8] . While low-molecular weight synthetic dyes provide advantages such as simplicity of use and high dynamic range (Δ F / F ratio), genetically encoded sensors offer high specificity, reversibility, subcellular targeting and transgenic options [9] . For these reasons genetically encoded H 2 O 2 probes have been successfully used in a number of contexts ranging from subcellular compartments of cells to tissues of living animals. The two types of genetically encoded probes for H 2 O 2 with superior performance in vivo are HyPer family reporters [5] , [6] , [8] and roGFP2-Orp1 (ref. 7) [7] . HyPer, together with its sequels HyPer-2 and HyPer-3, is a product of integration of a circular permutant of yellow fluorescent protein (cpYFP) into the regulatory domain of the bacterial H 2 O 2 sensing protein OxyR (OxyR-RD) [5] . Selectivity of OxyR-RD and HyPer towards H 2 O 2 is determined by a single Cys199 residue having two features: it has low pKa and resides in a hydrophobic pocket [10] , [11] , [12] . Low pKa makes the Cys199 redox active and the hydrophobic pocket precludes penetration of charged oxidants such as superoxide [11] . When oxidized, thiolate of Cys199 becomes repelled by the pocket to a close proximity to Cys208 residue and forms a disulfide bridge. Disulfide formation initiates conformational changes of the domain allowing DNA binding of the OxyR [11] and ratiometric changes in the excitation spectrum of HyPer 5 . roGFP2-Orp1 sensor uses oxidation of cysteines in roGFP2 by yeast Orp1 peroxidase [7] . Both roGFP and HyPer are green fluorescent proteins. The same is true for most of the single-fluorophore based sensors. These spectral characteristics of the available sensors preclude their application in combination with many other probes because of spectral overlaps. This issue could be addressed by expanding the spectral range of the genetically encoded redox probes to the red part of the visible spectrum. Sensors based on a circularly permuted red fluorescent proteins were not reported until recently when a breakthrough report from Campbell’s group described a palette of GECOs—genetically encoded Ca 2+ probes, based on cpFPs of different colours, including a red one [13] . We found that the simple technology used for high-throughput screening of GECO variants in E. coli colonies can also be applied for H 2 O 2 sensor screening. As a result, we produced HyPerRed, the first red fluorescent genetically encoded redox probe. Generating HyPerRed To generate a red fluorescent sensor for hydrogen peroxide, we initially replaced the cpYFP portion of HyPer with different circularly permuted red fluorescent proteins (FPs) based on mKate [14] and FusionRed [15] as well as cpRed, a circularly permuted red fluorescent protein mApple from the genetically encoded fluorescent sensor for calcium R-GECO1 (ref. 13) [13] . We prepared several semi-random expression libraries, which varied in the length of amino-acid linkers between the cpFP and two flanking OxyR-RD parts of the sensor. In each library, the sequences of the linkers were randomized to find unique variants with the best cpFP folding and maturation. Initially, we examined libraries of the sensor variants having either both linkers of two amino-acid (a.a.) length (as in R-GECO1) or having the first and the second linker three and two a.a. long, respectively (as in HyPer). To find the clones responding to H 2 O 2 , we acquired an image of the library on the plate under the fluorescent binocular microscope, sprayed an aerosol of 200 μM H 2 O 2 over the plates and then acquired a second image of the same plate. Determining the ratio of intensities in image 2 to image 1 should reveal the clones with H 2 O 2 -induced fluorescence increase (for ratios >1) or decrease (for ratios <1) of the signal. All examined libraries demonstrated poor fluorescent protein maturation at 37 °C with no clones responding to H 2 O 2 . Adding one a.a. to the second linker, we produced another set of libraries where both of the linkers were three a.a. in length. These libraries provided many clones efficiently maturating at 37 °C; however, only the libraries based on cpRed from R-GECO1 contained many clones responding to H 2 O 2 addition. The best of the detected clones corresponded to a protein that carried the linkers Pro-Arg-Thr and Ala-Gly-Val and that demonstrated an 80% increase in fluorescence upon H 2 O 2 addition; this protein was designated as HyPerRed ( Supplementary Fig. 1 ). HyPerRed characterization To characterize spectral properties and sensitivity of HyPerRed, we purified the protein using metal-affinity chromatography. To keep protein Cys residues reduced, we added 2 mM 2-mercaptoethanol (2-ME) to the extraction solution. Both 2-mercaptoethanol and imidazole used for elution of the protein were removed by gel filtration before spectroscopic measurements. 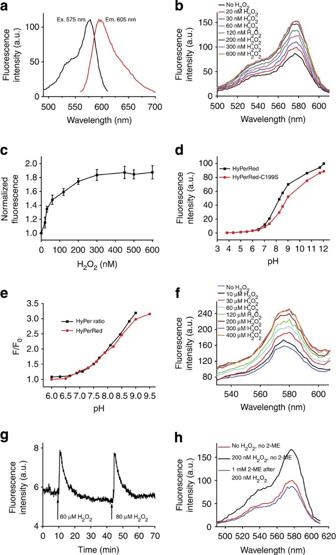Figure 1: Spectral properties and H2O2sensitivity of HyPerRed. (a) Excitation and emission spectra of purified HyPerRed. (b) Excitation spectrum of 15 nM HyPerRed in Tris-HCl (pH 7.5), 150 mM NaCl, 0.5 mM 2-mercaptoethanol, upon addition of indicated concentrations of H2O2. Emission was measured at 620 nm. (c) Increase in purified HyPerRed brightness (values±s.d., from five experiments) as a function of extracellular H2O2concentration. Values of 575 nm excitation were normalized to the value corresponding to zero H2O2. (d) pH dependency of isolated oxidized HyPerRed versus HyPerRed-C199S. (e) pH dependency of HyPerRed versus HyPer in the cytoplasm of eukaryotic cells. (f) Excitation spectrum of HyPerRed inE. colicell suspension upon addition of indicated concentrations of H2O2. Emission was measured at 620 nm. (g) Kinetics of fluorescence (excitation at 570 nm, emission at 620 nm) of HyPerRed inE. colicell suspension in response to successive addition of two pulses of H2O2. (h) Addition of 1 mM 2-mercaptoethanol to the oxidized HyPerRed leads to a reduction of the probe. Figure 1a shows fluorescence spectra of the purified HyPerRed. The sensor has an excitation peak at 575 nm and an emission peak at 605 nm. Titration of the probe against increasing concentrations of H 2 O 2 ranging from 10 to 600 nm demonstrated a response minimum at 20 nM and saturation at 300 nM ( Fig. 1b,c ). These results show that HyPerRed has the same sensitivity as green fluorescent versions of the sensor [6] . Figure 1: Spectral properties and H 2 O 2 sensitivity of HyPerRed. ( a ) Excitation and emission spectra of purified HyPerRed. ( b ) Excitation spectrum of 15 nM HyPerRed in Tris-HCl (pH 7.5), 150 mM NaCl, 0.5 mM 2-mercaptoethanol, upon addition of indicated concentrations of H 2 O 2 . Emission was measured at 620 nm. ( c ) Increase in purified HyPerRed brightness (values±s.d., from five experiments) as a function of extracellular H 2 O 2 concentration. Values of 575 nm excitation were normalized to the value corresponding to zero H 2 O 2 . ( d ) pH dependency of isolated oxidized HyPerRed versus HyPerRed-C199S. ( e ) pH dependency of HyPerRed versus HyPer in the cytoplasm of eukaryotic cells. ( f ) Excitation spectrum of HyPerRed in E. coli cell suspension upon addition of indicated concentrations of H 2 O 2 . Emission was measured at 620 nm. ( g ) Kinetics of fluorescence (excitation at 570 nm, emission at 620 nm) of HyPerRed in E. coli cell suspension in response to successive addition of two pulses of H 2 O 2 . ( h ) Addition of 1 mM 2-mercaptoethanol to the oxidized HyPerRed leads to a reduction of the probe. Full size image Cys199 is a critical residue reacting with H 2 O 2 and forming disulfide with Cys208 in both wtOxyR and HyPer. To prove that the same residue mediates HyPerRed response to H 2 O 2 , we substituted Cys199. While showing the same spectral properties as HyPerRed, HyPerRed-C199S was not sensitive to H 2 O 2 . Fluorescence of the majority of FPs varies with changes of pH. We measured pH dependence of HyPerRed ( Fig. 1d ). The pH titration curve of oxidized HyPerRed was similar to the titration curve of R-GECO in calcium-bound state [13] , with pKa of 8.5. pKa of HyPerRed-C199S (resembling fully reduced HyPerRed) was 8.7 ( Fig. 1d ). pH titration profiles of HyPerRed and HyPer in eukaryotic cells in the presence of nigericin and monensin were almost identical ( Fig. 1e ), although we were not able to calibrate at the pH values above 9 due to changes in the cell integrity. To evaluate the brightness of the sensor, we measured its extinction coefficient and quantum yield. The quantum yield of the purified oxidized HyPerRed was 0.29 remaining unchanged when the probe is reduced by 2-ME. The extinction coefficient of the oxidized probe at 577 nm was 39,000 M −1 cm −1 , giving brightness (a product of extinction coefficient and quantum yield) of 11,300, thus making the sensor more than fivefold brighter than HyPer ( Supplementary Table 1 ). Next we examined the sensitivity to external hydrogen peroxide of the HyPerRed expressed in the cytoplasm of E. coli cells. We suspended bacterial cells in PBS and measured their fluorescence spectra before and after the addition of hydrogen peroxide to a final concentration 10–400 μM. The minimal response of the probe was detected at 10 μM of hydrogen peroxide ( Fig. 1f ), which is close to the concentration required to activate HyPer and wild-type OxyR in vivo [6] , [9] , [10] . A volume of 300 μM of H 2 O 2 saturated the sensor ( Fig. 1f ). Oxidation of HyPerRed is reversible: after complete oxidation, the probe is reduced within 8–10 min and becomes available for a new cycle of oxidation ( Fig. 1g ). Being oxidized in vitro , HyPerRed can be reduced by 2-ME ( Fig. 1h ). HyPer is selective for H 2 O 2 and does not react with other oxidants [5] . However, changing the FP part of the sensor may lead to changes in the OxyR-RD part of the probe, potentially reducing its selectivity. To examine HyPerRed selectivity, we performed in vitro tests incubating HyPerRed with other oxidants ( Table 1 ). NO (produced by 1 mM MAHMA-NONOate), 1 mM oxidized glutathione (GSSG), superoxide anion radical (produced by xanthine—xanthine oxidase—catalase mixture) or peroxinitrite (SIN-1—catalase mixture) did not affect fluorescence of HyPerRed, indicating that HyPerRed retains the selectivity of the OxyR and HyPer proteins towards H 2 O 2 . Table 1 Effect of various oxidants on HyPer. Full size table Performance of HyPerRed in cultured mammalian cells We studied the reaction to hydrogen peroxide of HyPerRed expressed in the cytoplasm of a HeLa Kyoto culture using fluorescence microscopy. To evaluate the sensitivity of the sensor, we added increasing concentrations of H 2 O 2 to the imaging medium. Addition of 6 μM hydrogen peroxide induced small but detectable changes in fluorescence intensity of the sensor, similar to results obtained for the probe in the cytoplasm of the E. coli cells and similar to the results obtained with green HyPer versions. A volume of 200 μM H 2 O 2 led to maximal response ( Fig. 2 ). Therefore, HyPerRed appears suitable for H 2 O 2 detection in mammalian cells. 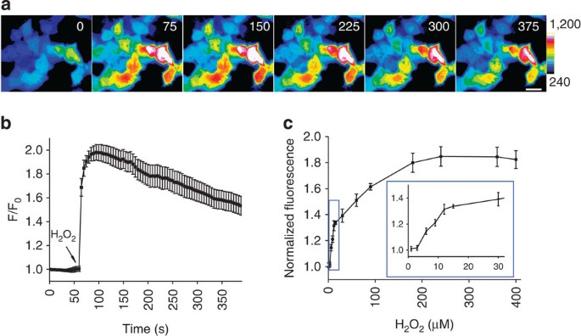Figure 2: HyPerRed responds to external H2O2in mammalian cells. (a) Images of HyPerRed in transiently transfected HeLa Kyoto cells exposed to 150 μM of H2O2at 60 s between the first and second picture. Numbers indicate timing in seconds. Scale bar, 40 μm. Lookup table indicates HyPerRed brightness change. (b) Timing of H2O2induced fluorescence change in the cells expressing HyPerRed shown on panela. Arrow indicates a time point of H2O2addition (1 min). (c) Increase in HyPerRed brightness in HeLa Kyoto cells as a function of extracellular H2O2concentration (values±s.d., 28 cells from three experiments). The inset shows the expanded area of the graph between zero and 30 μM H2O2. Figure 2: HyPerRed responds to external H 2 O 2 in mammalian cells. ( a ) Images of HyPerRed in transiently transfected HeLa Kyoto cells exposed to 150 μM of H 2 O 2 at 60 s between the first and second picture. Numbers indicate timing in seconds. Scale bar, 40 μm. Lookup table indicates HyPerRed brightness change. ( b ) Timing of H 2 O 2 induced fluorescence change in the cells expressing HyPerRed shown on panel a . Arrow indicates a time point of H 2 O 2 addition (1 min). ( c ) Increase in HyPerRed brightness in HeLa Kyoto cells as a function of extracellular H 2 O 2 concentration (values±s.d., 28 cells from three experiments). The inset shows the expanded area of the graph between zero and 30 μM H 2 O 2 . Full size image Next we evaluated the kinetic parameters of HyPerRed in the cytoplasm of eukaryotic cells. Measurements were made using fast imaging of the HeLa Kyoto cells using special microscopic μ- slides IV to quickly replace the imaging solution, which contained no H 2 O 2 , with medium containing a given concentration of hydrogen peroxide [8] . The kinetic parameters of oxidation were the same for HyPer, HyPerRed and wtOxyR. The concentration of H 2 O 2 at the half-maximal (K ox ) reaction rate between the probe and H 2 O 2 for HyPerRed was 140 nM compared with 160 nM for HyPer, 290 nM for HyPer-2 and 260 nM for HyPer-3 (ref. 6 ) (given the 500-fold drop in [H 2 O 2 ] across the plasma membrane determined earlier [6] ; Supplementary Table 1 ). The pseudo-first order reaction rate constant ( K s ) was 3 × 10 5 M −1 s −1 for HyPerRed compared with 5 × 10 5 M −1 s −1 for HyPer 6 ( Supplementary Table 1 ). Reduction half-time of HyPerRed was higher than that of HyPer and close to the reduction half-time of HyPer2. HyPerRed C199S demonstrated no response to H 2 O 2 in mammalian cells (data not shown). HyPerRed detects low signalling amounts of H 2 O 2 We next asked whether HyPerRed can be used to assess intracellular redox signalling in vitro . HyPer is a suitable tool for detecting the low physiological concentrations of H 2 O 2 that are relevant for cell signalling. The superior sensitivity and kinetic properties of HyPerRed suggest that this probe will also be able to detect small changes in [H 2 O 2 ] in mammalian cells upon growth factor stimulation. Addition of 100 ng ml −1 EGF to HeLa cells led to intracellular H 2 O 2 production and an increase in HyPerRed fluorescence ( Supplementary Fig. 2 , Supplementary Video 1 ) consistent with previous observations made using green versions of the probe [16] , [17] , [18] . Notably, HyPerRedC199S demonstrated no response to EGF in HeLa cells, indicating that pH is not a cause of HyPerRed spectral changes in this model (data not shown). Therefore, HyPerRed sensitivity and dynamic range allow measuring low levels of H 2 O 2 involved in cell signalling. Imaging H 2 O 2 and GSH/GSSG dynamics in different compartments It has been widely accepted that changes in ROS are associated with changes in redox state of main cellular redox couples, such as reduced-oxidized glutathione (GSH/GSSG) or NADP + /NADPH. Indeed, the cellular antioxidant machinery uses reduced forms of these couples to reduce thiols oxidized by H 2 O 2 . However, this notion has been recently challenged by studies of tissue- and organelle-specific age-dependent differences in the redox state of Drosophila melanogaster [19] . In particular, it was demonstrated that levels of H 2 O 2 may vary significantly without detectable changes in the GSH/GSSG balance. Mitochondria are one of the cellular compartments of continuous oxidative load. It is often stated, particularly in reviews [20] , that up to 1–2% of molecular oxygen consumed by the mitochondria undergo incomplete reduction in multiple sites of mitochondrial respiratory chain. However, such high ROS production has been detected only in vitro in isolated mitochondrial preparations [21] . The data on more complex settings such as cell cultures are often controversial, as they use mitochondrial or cytoplasmic ROS-detecting dyes, which are non-specific and phototoxic [22] , [23] . Experiments with mitochondria-targeted genetically encoded redox probes are still missing for most of the experimental models. Mitochondrial ROS production is often linked to cellular Ca 2+ signalling [24] . There is a general notion that Ca 2+ load stimulates mitochondrial ROS increase. There is a large body of evidence showing either increase [25] , [26] , [27] or decrease [28] , [29] , [30] in mitochondrial ROS production upon Ca 2+ load. However, these data were obtained using isolated mitochondria, and it remains unknown to what extent these observations can be extrapolated to mitochondrial ROS production in situ. Can this ROS production be detected using genetically encoded redox probes targeted to mitochondrial matrix? Would H 2 O 2 production in the matrix be associated with concomitant changes in GSH/GSSG ratio? Will the changes in the mitochondrial ROS production, if any, spread to the cytoplasm? To address these issues, we took an advantage of simultaneous imaging of red H 2 O 2 sensor and green fluorescent sensors for H 2 O 2 , pH and GSH/GSSG. First, we targeted HyPerRed to mitochondrial matrix by adding double mitochondrial localization sequence to its N terminus similar to dmito-HyPer, a mitochondrially targeted HyPer sensor [5] . Then we coexpressed HyPerRed-mito in HEK-293 cells with a variety of green redox biosensors targeted to either mitochondria or cytoplasm to detect changes in H 2 O 2 , GSH/GSSG and pH simultaneously. We used two methods to increase intracellular Ca 2+ levels: stimulation of cells with ATP, an agonist of purinergic receptors [31] , or with thapsigargin (TG), an inhibitor of SERCA Ca 2+ pump responsible for reuptake of calcium ions from the cytoplasm to the endoplasmic reticulum (ER) [32] . Both compounds induced marked increase of Ca 2+ in the cytoplasm ( Supplementary Fig. 3a,c ). Addition of ATP to HEK-293 cells did not lead to detectable changes in mitochondrial ROS production ( Supplementary Fig. 4 ). However, on addition of TG, we observed a small but well-defined peak of H 2 O 2 production in the matrix ( Fig. 3a–c , Supplementary Video 2 ), which is quantified in Fig. 3d , lower trace. As HyPerRed has the same pH-sensitivity profile as yellow HyPer versions, we examined whether the HyPerRed-mito response to TG was H 2 O 2 -specific and was not due to TG-induced matrix alkalinization. For that, we coexpressed HyPerRed-mito with mitochondrially targeted HyPerC199S (SypHer-mito [33] ). Whereas HyPerRed-mito responded to TG by transient increase in fluorescence, SypHer-mito ratio (F500/F420) did not change, indicating no changes in the matrix pH on TG addition ( Fig. 3c,d , Supplementary Video 3 ). This indicates that HyPerRed-mito fluorescence change is due to an increase in H 2 O 2 production. To prove that the response of HyPerRed-mito to TG is not a HyPerRed-specific artefact, we confirmed TG-induced H 2 O 2 production using dmito-HyPer ( Fig. 3e ). 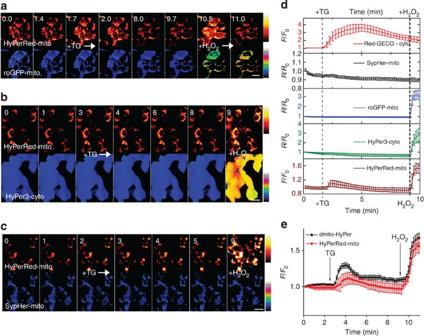Figure 3: Multiparameter imaging of H2O2, GSH/GSSG, Ca2+and pH. (a) Inhibition of SERCA Ca2+pump by TG induces temporal H2O2increase in the mitochondrial matrix, whereas GSH/GSSG ratio remains unchanged. HEK-293 cells were co-transfected with HyPerRed-mito (upper row) and roGFP-mito (lower row). Numbers indicate timing in minutes. Scale bar, 20 μm. Lookup tables indicate HyPerRed brightness (3,700 to 25,000, 16 bit scale) and roGFP-mito ratio (0.5 to 4). (b) H2O2does not spread from the mitochondria to the cytoplasm of the cells. HEK-293 cells were co-transfected with HyPerRed-mito (upper row) and HyPer3-cyto (lower row). Numbers indicate timing in minutes. Scale bar, 30 μm. Lookup tables indicate HyPerRed brightness (3,700 to 25,000, 16 bit scale) and HyPer-3 ratio (0.5 to 6). (c) Mitochondrial pH remains stable upon SERCA Ca2+pump inhibition and matrix H2O2release. HEK-293 cells were co-transfected with HyPerRed-mito (upper row) and SypHer-mito (lower row). Numbers indicate timing in minutes. Scale bar, 40 μm. Lookup tables indicate HyPerRed brightness (3,700 to 25,000, 16 bit scale) and SypHer ratio (0.5 to 4). (d) TG induces temporal H2O2increase in the mitochondrial matrix (measured using HyPerRed-mito), while cytosolic H2O2(HyPer3-cyto), mitochondrial GSH/GSSG (roGFP-mito) and mitochondrial pH (SypHer-mito) remain stable. In each experiment, HyPerRed-mito was co-expressed with either HyPer3-cyto or roGFP-mito or SypHer-mito. The panel shows values±s.d. for more than 100 cells in two or more experiments for each sensor combination. The agonist was added at a 1.7-min time point. For sample images see panels (a–c). (e) Similar to HyPerRed-mito, dmito-HyPer shows TG-induced matrix H2O2production, confirming specificity of HyPerRed signal. TG was added at a 2.5-min time point. Figure 3: Multiparameter imaging of H 2 O 2 , GSH/GSSG, Ca 2+ and pH. ( a ) Inhibition of SERCA Ca 2+ pump by TG induces temporal H 2 O 2 increase in the mitochondrial matrix, whereas GSH/GSSG ratio remains unchanged. HEK-293 cells were co-transfected with HyPerRed-mito (upper row) and roGFP-mito (lower row). Numbers indicate timing in minutes. Scale bar, 20 μm. Lookup tables indicate HyPerRed brightness (3,700 to 25,000, 16 bit scale) and roGFP-mito ratio (0.5 to 4). ( b ) H 2 O 2 does not spread from the mitochondria to the cytoplasm of the cells. HEK-293 cells were co-transfected with HyPerRed-mito (upper row) and HyPer3-cyto (lower row). Numbers indicate timing in minutes. Scale bar, 30 μm. Lookup tables indicate HyPerRed brightness (3,700 to 25,000, 16 bit scale) and HyPer-3 ratio (0.5 to 6). ( c ) Mitochondrial pH remains stable upon SERCA Ca 2+ pump inhibition and matrix H 2 O 2 release. HEK-293 cells were co-transfected with HyPerRed-mito (upper row) and SypHer-mito (lower row). Numbers indicate timing in minutes. Scale bar, 40 μm. Lookup tables indicate HyPerRed brightness (3,700 to 25,000, 16 bit scale) and SypHer ratio (0.5 to 4). ( d ) TG induces temporal H 2 O 2 increase in the mitochondrial matrix (measured using HyPerRed-mito), while cytosolic H 2 O 2 (HyPer3-cyto), mitochondrial GSH/GSSG (roGFP-mito) and mitochondrial pH (SypHer-mito) remain stable. In each experiment, HyPerRed-mito was co-expressed with either HyPer3-cyto or roGFP-mito or SypHer-mito. The panel shows values±s.d. for more than 100 cells in two or more experiments for each sensor combination. The agonist was added at a 1.7-min time point. For sample images see panels ( a – c ). ( e ) Similar to HyPerRed-mito, dmito-HyPer shows TG-induced matrix H 2 O 2 production, confirming specificity of HyPerRed signal. TG was added at a 2.5-min time point. Full size image H 2 O 2 generation can activate the antioxidant machinery, which relies in part on the cellular GSH pool. Therefore, one could expect that an increase in H 2 O 2 is associated with some decrease in GSH/GSSG ratio. To determine whether the TG-induced H 2 O 2 changes are associated with modulation of the redox state of thiols, we coexpressed HyPerRed-mito with mitochondrially targeted Grx1-RoGFP2 (roGFP-mito), a genetically encoded sensor for GSH/GSSG ratio [19] , [34] . While both of the probes responded very well to external saturating H 2 O 2 , TG only induced changes in HyPerRed-mito fluorescence but not in roGFP-mito, indicating no decrease in the GSH/GSSG ratio in the matrix ( Fig. 3a,d , Supplementary Video 2 ). The mitochondrial inner membrane is permeable to H 2 O 2 , as externally added oxidant was able to induce immediate changes in HyPerRed-mito, roGFP-mito ( Fig. 3a,d ) and dmito-HyPer ( Fig. 3e ) fluorescence. This suggests that TG-induced H 2 O 2 detected in the matrix using HyPerRed-mito could spread to the cytoplasm, or even that H 2 O 2 has a cytoplasmic origin and spreads to the matrix. To define the compartment responsible for the H 2 O 2 increase, we coexpressed HyPerRed-mito with non-targeted HyPer3 6 localized in the cytoplasm (HyPer3-cyto). HyPer3-cyto showed no changes on TG addition ( Fig. 3b,d , Supplementary Video 4 ), indicating that H 2 O 2 production has a mitochondrial origin and does not spread to the cytoplasm. Notably, the GSH/GSSG ratio in the cytoplasm remains stable as well (data not shown). Removing Ca 2+ from the media did not significantly affect the amplitude of the TG-induced H 2 O 2 peak ( Fig. 4a ), consistent with a previous observation that depleting Ca 2+ does not completely prevent TG-induced Ca 2+ rise in the cytoplasm, but makes it more transient [35] . Rotenone, an inhibitor of the respiratory chain Complex I, attenuated the H 2 O 2 increase ( Fig. 4a ), indicating the mitochondrial respiratory chain as a source of the oxidant. 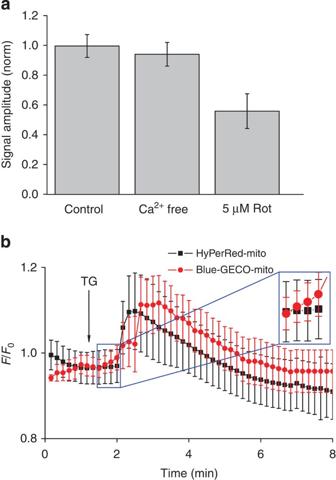Figure 4: TG-induced H2O2is produced by the mitochondrial respiratory chain. (a) Effects of Ca2+-free media and rotenone on the intensity of H2O2increase in mitochondria. The bars show normalized values±s.d., 25 cells from two experiments for Ca2+-free media, 42 cells from three experiments for rotenone. (b) Timing of mitochondrial H2O2production (HyPerRed-mito) compared with mitochondrial Ca2+elevation (B-GECO-mito). The curves were ‘synchronized’ by the TG addition time point (1 min). The inset shows the moment when mitochondrial Ca2+starts increasing before H2O2. Figure 4: TG-induced H 2 O 2 is produced by the mitochondrial respiratory chain. ( a ) Effects of Ca 2+ -free media and rotenone on the intensity of H 2 O 2 increase in mitochondria. The bars show normalized values±s.d., 25 cells from two experiments for Ca 2+ -free media, 42 cells from three experiments for rotenone. ( b ) Timing of mitochondrial H 2 O 2 production (HyPerRed-mito) compared with mitochondrial Ca 2+ elevation (B-GECO-mito). The curves were ‘synchronized’ by the TG addition time point (1 min). The inset shows the moment when mitochondrial Ca 2+ starts increasing before H 2 O 2 . Full size image Addition of TG to the cells induces a rapid increase of Ca 2+ in the cytoplasm followed by delayed and small rise of mitochondrial Ca 2+ ( Supplementary Fig. 3b,d ). Mitochondrial H 2 O 2 generation coincided with Ca 2+ increase in the matrix ( Fig. 4b ). The frame rate of 0.1 Hz and the dynamic range of the probes did not allow to draw unequivocal conclusions about the temporal sequence of these events, but we observed the Ca 2+ increase in the matrix usually 10–20 s before the increase in the H 2 O 2 signal. The lack of HyPer3-cyto oxidation in the cytoplasm on TG addition to the cells argues against the concept that mitochondrial H 2 O 2 has a signalling role in the cytoplasm, at least in our experimental system. Rather, these results suggest that matrix H 2 O 2 can act as a signal at the level of mitochondria. However, there remains a possibility of H 2 O 2 leaking from matrix to the mitochondrial intermembrane space (IMS). IMS by itself can be an origin of ROS, originating from Complex III [36] . We therefore asked whether the H 2 O 2 signal induced by TG exists in the IMS. For that, we fused HyPer2 with SMAC/DIABLO protein [37] to direct the fusion protein to the IMS and co-transfected HyPer2-IMS with HyPerRed-mito into the HEK-293 cells. Both sensors demonstrated mitochondrial staining. To show that HyPer2-IMS localizes to the IMS, we used a simple mitochondrial uncoupler test. As the matrix of energized mitochondria is more alkaline than IMS/cytoplasm, we could expect acidification of the matrix on addition of an uncoupler (CCCP) to the cells. Therefore, if HyPer2 or HyPerRed is localized in the matrix, HyPer2 ratio or HyPerRed brightness would decrease upon CCCP addition. In contrast, IMS has either the same pH as the cytoplasm due to rapid proton exchange via mitochondrial outer membrane or is slightly more acidic due to the proton gradient across the inner mitochondrial membrane. Therefore, the probes in the IMS would show either no change or an increase in ratio/brightness upon uncoupling of the electron transport chain. Indeed, 36 h post transfection HyPer2-IMS did not respond to CCCP, whereas HyPerRed-mito did ( Fig. 5a ), indicating complete separation of the sensors across the mitochondrial inner membrane. Addition of TG induced an increase of HyPerRed-mito fluorescence as shown before ( Fig. 3 ), but did not affect HyPer2-IMS ratio ( Fig. 5 ). This is indicative of the absence of IMS-specific ROS generation or of the spread of H 2 O 2 from the matrix to the IMS upon blocking ER Ca 2+ uptake via SERCA. 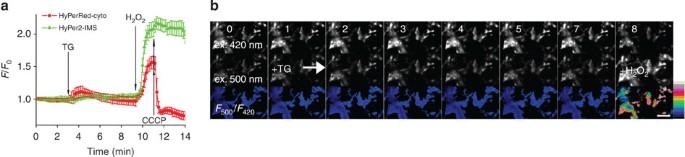Figure 5: H2O2does not spread from the mitochondrial matrix to the IMS. (a) H2O2produced in the mitochondrial matrix (HyPerRed-mito) does not spread to IMS (HyPer2-IMS). TG was added at a 3-min time point. The panels show values±s.d., more than 20 cells in two experiments. (b) Images of HyPer-2-IMS in transiently transfected HEK-293 cells exposed to TG. Numbers indicate timing in minutes. Scale bar, 60 μm. Lookup table indicates HyPer-2-IMS ratio change (0.5–6). Figure 5: H 2 O 2 does not spread from the mitochondrial matrix to the IMS. ( a ) H 2 O 2 produced in the mitochondrial matrix (HyPerRed-mito) does not spread to IMS (HyPer2-IMS). TG was added at a 3-min time point. The panels show values±s.d., more than 20 cells in two experiments. ( b ) Images of HyPer-2-IMS in transiently transfected HEK-293 cells exposed to TG. Numbers indicate timing in minutes. Scale bar, 60 μm. Lookup table indicates HyPer-2-IMS ratio change (0.5–6). Full size image Taken together, our results show that inhibition of Ca 2+ reuptake into the ER induces small, local and transient increase in matrix H 2 O 2 production, which is not accompanied with detectable GSH oxidation. Furthermore, they indicate that H 2 O 2 does not spread from the matrix to the IMS or the cytoplasm. Genetically encoded fluorescent probes offer a unique opportunity to study cellular events in the most native environment without harm for the cells and tissues. Single-fluorophore probes based on circularly permuted fluorescent proteins have advantages of relatively low-molecular weight compared with fluorescence resonance energy transfer (FRET)-based sensors and of high dynamic range [5] , [38] . Their working range occupies a narrow part of the spectrum allowing multiparameter imaging simultaneously with other fluorophores. When developing the HyPer probe, we designed a simple strategy of integration of cpFP into a flexible region of a sensitive domain (OxyR-RD in case of HyPer), which allows generation of a probe by combining as few as two proteins. This principle was further used to make sensors for detecting ADP:ATP ratio [39] , NADH:NAD + ratio [40] and glutamate [41] . However, until recently, all of the circularly permuted FPs were green emitters. A few examples of red fluorescent permuted proteins reported have not been used in currently available sensors [42] . Seminal work of Campbell and coworkers [13] resulted in the first genetically encoded cpFP-based Ca 2+ sensors occupying a wide range of visible colours, from blue to red. Red fluorescent proteins and RFP-based sensors are important for in vivo imaging, as the tissue penetration of the light increases with the increase in wavelength. A simultaneous monitoring of different processes in living cells and tissues using microscopy, known as multiparameter imaging, needs chromophores with non-overlapping spectra. We substituted cpYFP in HyPer to cpRFP from R-GECO1 probe and utilized high-throughput screening of the E.coli libraries to find optimal variants of the red HyPer. While selecting for fast-maturing probes, we found that the library in which the length of both of the linkers between OxyR-RD and cpRFP were three a.a. provided the maximal number of clones with fluorescent proteins maturating at 37 °C. Efficient maturation indicates that the OxyR-RD part of the sensor does not notably perturb the structure of the FP and we can suggest that conversely the cpRFP region does not distort significantly the H 2 O 2 -sensing domain. The length of the linkers flanking cpRFP in R-GECO is two a.a. for both. Therefore, the length and composition of the linkers appear to be unique for each sensor based on the particular cpFP. This was not expected, as linkers SAG and GT flanking cpYFP in Ca 2+ sensing Pericam [38] were found to be optimal for the similar cpYFP in HyPer 5 . Unfortunately, there is still no clear rationale for the linker design. Varying the linker length followed by the random mutagenesis of the linkers is still the most efficient way to couple cpFP with the sensitive domain. Fluorescence of HyPer depends on pH [5] . Therefore, HyPer-C199S control or other control for pH should be used in parallel experiments. Unfortunately, the pKa of cpmApple used in R-GECO1 and HyPerRed is the same as for HyPer and their pH-titration profiles are similar. We therefore strongly recommend using HyPerRed-C199S or HyPer-C199S as a control for pH changes in parallel experiments. HyPerRed is intensiometric, that is, it is a single wavelength sensor and not ratiometric as HyPer. Ratiometricity has several advantages such as compensation for movement artefacts, independence of protein expression level variability and possibility to calibrate the probe against the concentration of the molecule measured. However, ratiometric probes occupy wider spectral range, limiting possible combinations of the probes in multiparameter imaging. Moreover, ratiometricity, if needed, can be reached by fusing the sensor with FP of different colour (example is an NAD/NADH sensor Peredox [40] ) or using spectrally distinct FP as a volumetric control. Kinetics of the reaction of HyPerRed with H 2 O 2 is similar to that of HyPer and OxyR, indicating that insertion of the new cpRFP instead of cpYFP in HyPer does not perturb OxyR-RD function. The sensitivity for all HyPer probes is also similar with K ox between 140 nM (HyPerRed) and 290 nM (HyPer-2). The dynamic range of HyPerRed is ~30% lower compared with HyPer, but still large enough to detect small amounts of growth factor-induced H 2 O 2 in HeLa cells. Using HyPerRed, we were able, for the first time, to monitor both H 2 O 2 and GSH/GSSG or pH changes in real time within the same compartment. Targeting HyPerRed into the mitochondrial matrix in combinations with green-emitting mitochondrial and cytoplasmic probes for GSH/GSSG, H 2 O 2 and pH, we detected mitochondrial H 2 O 2 production associated with inhibition of Ca 2+ uptake to the ER. Surprisingly, extracellular ATP, which induces Ca 2+ transients of large amplitude, did not stimulate mitochondrial ROS production. This could be explained within a model where Ca 2+ exchange between cytoplasm and mitochondria takes place in the specialized subcompartments without involvement of the global cytosolic Ca 2+ pool. Increasing evidence indicates compartmentalization of Ca 2+ and redox signalling. Therefore, we favour the idea that TG acts at the level of local Ca 2+ domains between the mitochondria and the ER. Intuitively, it seems reasonable that an increase in ROS should be paralleled with a decrease in GSH/GSSG ratio, as GSH-based antioxidant systems utilize GSH to reduce oxidized thiols and to eliminate H 2 O 2 . At the same time, roGFP ratio changes are often misinterpreted as reflecting a ROS increase, while they in fact reflect thiol exchange between roGFP and cellular thiol pool [9] , [43] . We have shown, for the first time, that a small H 2 O 2 increase in the mitochondrial matrix does not cause any detectable change in the GSH/GSSG ratio. In contrast, addition of high amounts of external H 2 O 2 (100 μM) caused an immediate decrease of the GSH/GSSG levels in both mitochondria and cytoplasm. Our semi-quantitative estimate of the H 2 O 2 increase in the matrix indicates ~30–50 nM H 2 O 2 at the peak. Given that GSH concentrations within these compartments are in the millimolar range, it seems reasonable that the GSH/GSSG ratio remains stable. Our results are in agreement with previous experiments showing that in tissues of Drosophila melanogaster H 2 O 2 levels can vary much more than the GSH/GSSG ratio [19] . Another intriguing aspect of the TG-induced H 2 O 2 increase is its transient nature. SERCA inhibition causes an immediate increase in H 2 O 2 , but only for 10 min. This could be explained by compensatory mechanisms that sequestrate or pump out Ca 2+ from the sites responsible for TG-induced ROS increase. It may also be indicative of the transient signalling nature of H 2 O 2 . However, the target for this signal as well as the source of the oxidant remains unknown. The fact that blocking electron flow by rotenone abrogates TG-induced ROS increase points out respiratory chain as a source of H 2 O 2 . The absence of H 2 O 2 in the IMS and cytoplasm clearly indicates matrix origin of the oxidant. However, a specific site that is responsible for TG-induced electrons leaks to molecular oxygen remains to be determined. Ca 2+ deregulation, particularly in the ER, is associated with many pathological states extensively reviewed in the literature [44] . Therefore, H 2 O 2 production caused by SERCA inhibition could be a part of pathology progression. However, the transient nature of the H 2 O 2 rise shows that eukaryotic cells can resist ER stress, at least to some extent. What would be the next steps in red fluorescent sensor development towards ideal probes, including those for redox events? The best probe should be bright, pH-stable, red-excitable (or, better, far-red-excitable) and red or far-red emitting. pH stability is very important as pH changes accompany many intracellular events, especially in endo- and lysosomal compartments and in the mitochondrial matrix. We expect that use of circular permutations of RFPs with low pKa, such as mKate (pKa 5.4) or FusionRed (pKa 4.6), may solve this problem. One of the disadvantages of the green probes is their limited performance in many in vivo models because of poor tissue penetration of violet or blue excitation light and green emitted light [45] . Brightness and long wavelength spectra would be especially appreciated in an in vivo imaging in non-transparent tissues, such as the mouse brain, where the depth of the light penetration and light scattering/absorption by the tissue are the critical parameters affecting the quality of imaging. Whereas the brightness of the probe can be improved using random or site-directed mutagenesis, the advance towards the far-red spectrum is more complicated, as GFP-like proteins seem to have a limited capacity to be spectrally shifted. A promising alternative is to use far-red fluorescent proteins based on phytochromes [46] , [47] , [48] . The first reported versions of such proteins are dimeric and have low quantum yield and brightness, but their further improvement together with a search for splitting/permutation sites within them could make them an ideal platform for the in vivo sensors. Taken together, our results present a first significant step in shifting redox probes towards the red spectrum. Now H 2 O 2 can be imaged in parallel with a large variety of messengers, metabolites and enzymatic activities as reported with blue-to-yellow emitting genetically encoded probes, CFP-YFP or BFP-GFP FRET sensors and various synthetic dyes. Generation of libraries and cloning Tersus polymerase (Evrogen) was used for non-mutagenic PCR amplifications. The original HyPer 5 and Red-GECO [13] plasmids were used as a template DNA for PCR. Fragments encoding N- and C-terminal parts of OxyR-RD and cpRed with random linkers were mixed in equal amounts and used in the ‘overlap extension’ PCR for combining into a whole construct. The full-length product was purified by agarose gel electrophoresis and then predigested PCR product was ligated into the target vector (pQE-30 or pC1). T4 ligase in Rapid Ligation Buffer (Promega) or T4 ligase (Evrogen) was used for ligation. The selection of clones expressing the full-length sensor variants was carried out using a fluorescent binocular microscope Olympus US SZX12. We captured an image of the library, sprayed 200 μM H 2 O 2 and then acquired the second image without moving the plate. Determining the ratio of intensities in image 2 to image 1 revealed the clones with H 2 O 2 -induced fluorescence increase. Conversely, determining the ratio of intensities in image 1 to image 2 indicated clones with inverse phenotype. Bacterial colonies with 80% increase of fluorescence to addition of hydrogen peroxide were picked to Petri dishes with LB-agar containing ampicillin. Spectral characteristics of selected clones were evaluated using a fluorescent spectrophotometer Varian Cary Eclipse. Bacterial cells were transferred from Petri dishes to 2 ml of PBS buffer (25 °C) in a plastic spectrofluorimeter cuvette. We detected excitation spectra in the range of 530–610 nm (emission at 630 nm) before and after addition of 10–300 μM H 2 O 2 to the cells. IMS-HyPer2 was produced by replacing the EGFP-coding region of IMS-EGFP by HyPer2-coding DNA from HyPer2-dMito vector using restriction enzymes BamHI and NotI. To produce HyPerRed-mito, we replaced sequence of Hyper in d-mitoHyPer pC1 plasmid (Evrogen) to HyPerRed one using Bam HI and Afe I sites Cell culture and transfection HeLa Kyoto (EMBL collection) or HEK-293 cells (ATCC) were seeded into 35-mm glass bottom dishes (MatTek) and cultured in DMEM with 10% FCS (PAA Laboratories) at 37 °C in a 5% CO 2 atmosphere. After 24 h, cells were transfected by a mixture of 1 ng DNA (or 0.65 ng DNA of each vector for co-transfection) and 3 μl (6 μl for co-transfection) X-treme GENE 9 transfection reagent per one dish. After 8–10 h, cell medium was replaced by fresh medium. For reaction rate experiments, HeLa-Kyoto cells were seeded into μ-slides VI (IBIDI) and transfected 24 h later by a mixture of DNA and X-treme GENE 9 transfection reagent. Stimulation of the cells Twenty-four hours after transfection, the HeLa Kyoto cells or HEK-293 cells were incubated for 2 h in HBSS supplemented with 20 mM of HEPES-NaOH pH 7.4 at 37 °C. The dishes were transferred onto the microscopic stage of a widefield fluorescent microscope (Leica DMI 6000 B) equipped with an HCX PL Apo CS 40.0 × 1.25 Oil UV objective. After 3–5 images acquired, 100 ng ml −1 EGF or 10 μM thapsigargin was added. Fluorescent imaging Microscopy of cells was carried out using Leica DMI6000 at 37 °C in HBSS supplemented with 20 mM of HEPES. For HyPerRed TX2 filter cube was used (excitation: BP 560/40, dichromatic mirror 595, emission: BP 645/75). Recording intervals were 5 s. To determine the response of the probe to H 2 O 2 , we added a solution of H 2 O 2 in 100 ml volume to the cells to a final concentration of 6–200 μM. The final processing of images was performed using the ImageJ software. [Ca 2+ ] i was determined using 1 μM Fura 2/AM, as described before [49] . The images were analysed using TILL Vision software. Protein expression and purification To purify HyPerRed competent E.coli XL1Blue cells were transformed with pQE30 plasmid harbouring HyPerRed gene. Single colonies selected on ampicillin were picked and used to inoculate 200 ml LB/ ampicillin medium (1 mg ml −1 ). Bacterial cultures were shaken at 200 r.p.m. for 24 h at 37 °C. Bacteria were harvested by centrifugation at 4,000 × g for 30 min (4 °C). The pellet was resuspended in 7 ml of buffer A (40 mM Tris-HCl, pH 7.5, containing 150 mM KCl, 10 mM MgSO4) with 2 mM 2-mercaptoethanol, lysed by ultrasound on blue ice bath for 20 min and clarified by centrifugation at 18,000 × g at 4 °C for 30 min. Proteins were purified from the cell-free extracts by metal-affinity chromatography (Talon Metal Affinity Resin, Clontech). A 3 ml of the cell-free extract was applied to a column filled with 3.5 ml resin equilibrated with buffer A containing 2-mercaptoethanol. The column was washed with 35 ml of buffer A with 2-mercaptoethanol and then the protein was eluted with buffer A with 200 mM imidazole. The purified protein was immediately applied to a 5 ml Sephadex G-25 column (GE Healthcare) equilibrated with buffer A to remove imidazole. Spectroscopic characterization of the probes As we were not able to isolate HyPerRed in completely reduced form, the molar extinction coefficient ( ε ) and the quantum yield (QY) were measured for the probes in the oxidized form. Equal aliquots of HyPer variants were diluted in PBS and their absorption spectra were measured in the range of 200–800 nm to determine molar extinction coefficients of proteins. The molar extinction coefficients were determined using the formula ε i=Absi*Cprot(M) −1 *l(cm) −1 where, Absi—the optical density at the absorption maximum and l—the optical path length. Concentrations of proteins were determined by Bradford protein assay, measuring protein concentration through absorption at 260–280 nm and by biuret protein assay. To determine the quantum yield of fluorescence of HyPerRed, the emission spectra of the fluorescence excited at 575 nm were measured and compared with the proteins with known QY (standards mKate2 and mCherry). QY for each protein was determined by using the formula QY=QY1*(Abs1*Em2*Abs2 −1 *Em1 −1 ) where Abs1 and Em1—the values of the absorption and emission of standard (mKate2: Abs588 Em633; mCherry: Abs 577 Em610), Abs2 and Em2—the values of the absorption (Abs575) and emission (Ex605) for HyPerRed variant, QY1—the quantum yield of fluorescence of standard (mKate2:0,62 and mCherry: 0,22), QY—the quantum yield of fluorescence of HyPerRed. To determine the apparent pKa buffers with pH values from 3 to 11.5 in 0.5 pH unit intervals were prepared. A solution containing 40 mM trisodium citrate and 40 mM borax was adjusted to pH 11.5 and HCl (12 and 1 M) was then added dropwise to provide solutions with needed pH values. The pH titration of oxidized protein was performed by adding 15 μl of concentrated protein in PBS into 2 ml of each of the buffers described above. The fluorescence of probe in each buffer condition was recorded using a spectrophotometer Varian Cary Eclipse. Selectivity and reaction rates of the probes Purified protein was kept on ice. In each experiment, we placed 3 ml of 25 nM HyPerRed in the buffer containing 25 mM Tris-HCl (pH 7.5), 150 mM NaCl into the plastic spectrophotometer cuvette. The fluorescence was recorded using a Varian Cary Eclipse spectrofluorimeter. After the initial fluorescence spectrum recording, various oxidants were added into the reaction buffer and the spectrum was recorded again immediately and every minute up to 15 min after addition of the oxidant. To produce superoxide anion, we used 30 mM xanthine and 25 mU xanthine oxidase. To exclude possibility of HyPerRed oxidation by H 2 O 2 generated by dismutation of superoxide anion, 100 mU catalase was added to the reaction buffer. The half-oxidation constant ( K ox ) and the rate constants ( K s ) of the reaction with H 2 O 2 were determined using fast imaging in the living cells. HeLa-Kyoto cells on μ-slides-VI (IBIDI) were imaged at high speed with fast cell medium change. H 2 O 2 was added at final concentration ranging from 6 to 400 μM (final concentration) to the separate tracks of μ-slides. The reaction rate (V) determined as Δratio/Δtime at the linear region of the curve. K ox was the concentration of H 2 O 2 at which reaction rate between HyPer and H 2 O 2 was the half of the maximum. The pseudo-first order reaction rate constants between HyPer variants and H 2 O 2 were determined as K s =V/[H 2 O 2 ]. Constructs availability: HyPerRed and HyPerRed-C199S are available from AddGene ( http://www.addgene.org/Vsevolod_Belousov/ ). How to cite this article : Ermakova, Y. G. et al. Red fluorescent genetically encoded indicator for intracellular hydrogen peroxide. Nat. Commun. 5:5222 doi: 10.1038/ncomms6222 (2014).